Molecular actuators driven by cooperative spin-state switching Molecular switches have great potential to convert different forms of energy into mechanical motion; however, their use is often limited by the narrow range of operating conditions. Here we report on the development of bilayer actuator devices using molecular spin crossover materials. Motion of the bilayer cantilever architecture results from the huge spontaneous strain accompanying the spin-state switching. The advantages of using spin crossover complexes here are substantial. The operating conditions used to switch the device can be manipulated through chemical modification, and there are many existing compounds to choose from. Spin crossover materials may be switched by diverse stimuli including light, temperature, pressure, guest molecules and magnetic field, allowing complex input combinations or highly specific operation. We demonstrate the versatility of this approach by fabricating actuators from four different spin crossover materials and by using both thermal variation and light to induce motion in a controlled direction. The development of actuator devices targeted at specific applications requires novel materials, the comprehension of their behaviour from macro- to nano-scale and the development of tools to process and operate them. At the most basic level, actuators convert a form of energy into motion. As we build ever smaller machines to perform tasks at the nano-scale, we must also develop the motors to power and control them. Recent important developments in this direction include nano-scale motors directed by light or chemical gradients capable of collective behaviour [1] and energy harvesting through stochastic motion of a single hydrogen molecule being used to drive a macroscopic mechanical oscillator [2] . Research in the field of molecular machines [3] , [4] , [5] , [6] has led to several encouraging prototypes in which molecular-scale motions could be amplified to produce macroscopic movement in a manner which may be understood by analogy to bimetallic strips [7] , [8] . Bimetallic strips are classically used to transduce thermal energy into motion and have been used for many years in thermometers and temperature sensors. They work on the basis of two different metals with different coefficients of thermal expansion strongly bonded together. The differential thermal expansion of the two layers causes the strip to bend when heated or cooled. The deliberate construction of a bimetallic strip analogue (BSA) designed to amplify motion produced by a phase transition has recently been demonstrated for VO 2 , which undergoes a thermally induced metal-insulator transition above room temperature, concomitant with a 0.3% volume change in the material [9] , [10] . Very recently, micro-actuators were also created from this same material, and actuation was observed as a direct result of the phase transition [11] . However, this system is restricted by the very narrow operating temperature range and relatively small volume change, severely limiting the potential applications of the actuating device. Similar limitations as to the switching conditions also apply to the molecular switches and machines mentioned above. If the BSA design is to be successfully scaled down to produce useful motion at reduced length scales, a significantly more versatile class of materials capable of specific motion, working in a wide variety of environmental conditions and in response to a range of different stimuli is needed. The change in material volume that accompanies the molecular switching between high-spin- (HS) and low-spin (LS) states during spin crossover (SCO) is usually around 5%, although values up to 13% have been observed for the [Fe(L){M(CN) 4 }] framework materials [12] . This is much higher than the differences of <1% shown to produce the dramatic macroscopic movement in the above examples. Furthermore, switching between HS and LS states is possible in response to several different external stimuli, revealing a very versatile transducer, potentially capable of converting many forms of energy into motion. The response of these systems to changes in the temperature, pressure, light irradiation, magnetic field, chemical species and so on should allow for complex combinations of input stimuli, increasing the scope of potential applications [13] . Another advantage of these systems is the hundreds of known SCO compounds available with a variety of active working ranges from cryogenic to well in excess of ambient temperature [14] , [15] . It is also interesting to note that the spin-state switching is often associated with hysteresis phenomena, implying a potential for shape-memory functions. SCO molecules would thus seem to be a perfect candidate for the development of micro- and macroscopic molecular machines, with properties that are highly tunable to the desired application. We report here on the successful fabrication of actuators from four different SCO materials, using both single crystal and composite bilayer architectures. The single-crystal BSAs are constructed from needle-like crystals of a three-dimensional (3D) coordination network coated in a thin layer of Al metal and suspended in a cantilever geometry. Cantilever deflections caused by thermal expansion and SCO are very different in magnitude and are opposite in direction, demonstrating unambiguously that the spin-state switching is capable of actuation using this approach. Both thermal variation and light irradiation were also used to induce SCO and thus motion in these single-crystal BSAs. In the case of the composite BSAs, three different SCO complexes are embedded in polymer films to act as the active layer, with a second inert polymer layer forming the bilayer structure. This simple and highly versatile approach allows the use of virtually any compound from the vast library of SCO complexes as the active layer. We have adapted traditional mechanical models to calculate the Young’s Modulus and estimate the forces generated by the actuator devices, allowing comparison with other actuating materials. Single crystals of {Fe(3-CNpy)[Au(CN) 2 ] 2 }· 2 3 H 2 O The thermal expansion properties of needle-like tetragonal crystals of the 3D SCO coordination polymer {Fe(3-CNpy)[Au(CN) 2 ] 2 }· 2 3 H 2 O ( 1 ), where py=pyridine, were investigated using variable temperature X-ray diffraction. A uniaxial negative thermal expansion (NTE) property of the crystals in the HS state was observed, where the long axis of the crystal (the crystallographic c axis) slightly increases on cooling from 290 to 130 K. Subsequently, the first-order HS→LS spin transition causes a substantial spontaneous strain (Δ c / c =0.01), ~10 4 times larger than the strain associated with thermal expansion in an equivalent range of temperature. The effect of SCO and NTE on the c axis of the crystal and illustrations of how the two phenomena affect the shape of the as-synthesized crystal are shown in Fig. 1 . The barely perceptible effect of NTE and SCO on the shape and size of the free crystals is shown in Supplementary Fig. S1 . Raman spectroscopy was used to identify spin-state markers for HS and LS states, as shown in Supplementary Fig. S2 . The thermal dependence of these modes is shown in Fig. 1c , clearly revealing an abrupt SCO with hysteresis as previously reported [16] , as well as a light-induced excited spin-state trapping (LIESST) effect at low temperature. 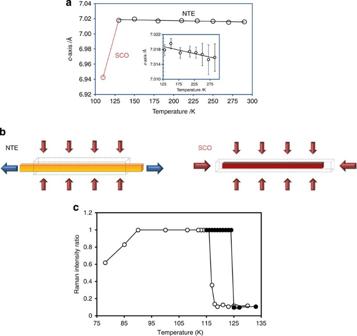Figure 1:NTE and SCO effects on the as-synthesized crystal. (a) Thermal dependence of the crystallographiccaxis on cooling from 290 to 110 K (open black circles are the HS state, open red circles are the LS state). The solid black and red lines serve as a guide to the eye for the effects of NTE and SCO, respectively. Thecaxis corresponds to the long axis of the needle-like crystal. Inset: close-up of the expansion in the HS state between 290 and 130 K. (b) Illustration of the effect of NTE and SCO on the crystal upon cooling. Arrows indicate the direction of length change. The dashed box represents the crystal shape before NTE or SCO and the coloured box after these processes. (c) Thermal dependence of the intensity ratio of the characteristic LS:HS Raman modes on a single crystal of1(open black circles are for cooling, closed black circles are for warming). Figure 1: NTE and SCO effects on the as-synthesized crystal . ( a ) Thermal dependence of the crystallographic c axis on cooling from 290 to 110 K (open black circles are the HS state, open red circles are the LS state). The solid black and red lines serve as a guide to the eye for the effects of NTE and SCO, respectively. The c axis corresponds to the long axis of the needle-like crystal. Inset: close-up of the expansion in the HS state between 290 and 130 K. ( b ) Illustration of the effect of NTE and SCO on the crystal upon cooling. Arrows indicate the direction of length change. The dashed box represents the crystal shape before NTE or SCO and the coloured box after these processes. ( c ) Thermal dependence of the intensity ratio of the characteristic LS:HS Raman modes on a single crystal of 1 (open black circles are for cooling, closed black circles are for warming). Full size image Bilayer actuators of {Fe(3-CNpy)[Au(CN) 2 ] 2 }· 2 3 H 2 O These highly anisotropic crystals were anchored to graphite rods with epoxy resin and were subsequently coated with a thin film of Al metal to produce freestanding composite cantilevers as shown in Fig. 2a . The effect of changing temperature on the cantilever shape was recorded between 343 and 78 K, as shown in Fig. 2 and Supplementary Movie 1 . The tip deflection as a function of temperature of the cantilever shown in Fig. 2 is plotted in Fig. 3a . The same effects were also reproduced on several other BSAs of 1 ( Supplementary Fig. S3 ). Figure 3b shows tip displacement of one of these cantilevers during several consecutive thermal cycles, revealing that both the displacement and observed hysteresis are stable to repeated thermal cycling. 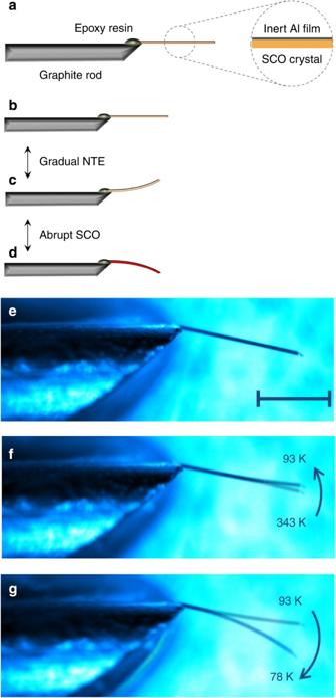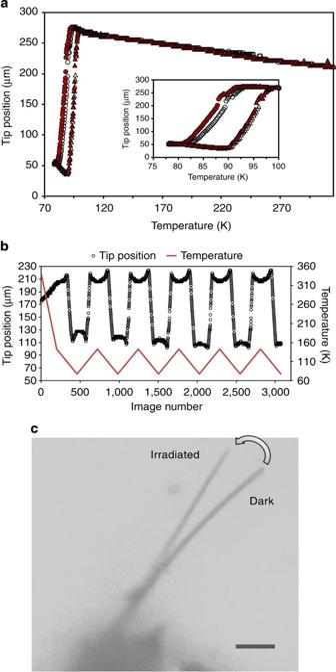Figure 3:Temperature- and light-induced actuation. (a) Tip position along a straight line as a function of temperature for the cantilever shown inFig. 2between 343 and 78 K. Open black circles are for the first cooling cycle, closed black circles are for the second cooling cycle, open black, triangles are for the first warming cycle, closed red triangles are for the second warming cycle. (b) Displacement of a second cantilever tip as a function of cycle number during repeated thermal cycling. (c) Effect of irradiation with a defocused laser beam (532 nm) on the deflection of a BSA of1at 4 K, scale bar represents 50 μm. Details of image treatment that yield data in (a,b) are provided in the Methods section. Heating and cooling rates were 5 K min−1(343–143 K) and 2 K min−1(143–78 K). Figure 2:Cantilever design and actuation in response to NTE and SCO. (a) Illustration of the composite structure of the cantilever. (b–d) Illustration of the effect of NTE and SCO on the cantilever (b—high-temperature HS,c—low-temperature HS andd—low-temperature LS). (e) Optical microscope image of the cantilever at 343 K. Scale bar represents 500 μm. (f) Comparison of the cantilever at 343 and 93 K, highlightling the deflection caused by NTE. (g) Comparison of the cantilever at 93 and 78 K, highlighting the SCO-induced actuation. Figure 2: Cantilever design and actuation in response to NTE and SCO . ( a ) Illustration of the composite structure of the cantilever. ( b – d ) Illustration of the effect of NTE and SCO on the cantilever ( b —high-temperature HS, c —low-temperature HS and d —low-temperature LS). ( e ) Optical microscope image of the cantilever at 343 K. Scale bar represents 500 μm. ( f ) Comparison of the cantilever at 343 and 93 K, highlightling the deflection caused by NTE. ( g ) Comparison of the cantilever at 93 and 78 K, highlighting the SCO-induced actuation. Full size image Figure 3: Temperature- and light-induced actuation . ( a ) Tip position along a straight line as a function of temperature for the cantilever shown in Fig. 2 between 343 and 78 K. Open black circles are for the first cooling cycle, closed black circles are for the second cooling cycle, open black, triangles are for the first warming cycle, closed red triangles are for the second warming cycle. ( b ) Displacement of a second cantilever tip as a function of cycle number during repeated thermal cycling. ( c ) Effect of irradiation with a defocused laser beam (532 nm) on the deflection of a BSA of 1 at 4 K, scale bar represents 50 μm. Details of image treatment that yield data in ( a , b ) are provided in the Methods section. Heating and cooling rates were 5 K min −1 (343–143 K) and 2 K min −1 (143–78 K). Full size image The LIESST effect observed in this sample meant that it was possible to induce reversible tip deflection at a single fixed temperature via light irradiation using a laser beam, as shown in Fig. 3c and Supplementary Fig. S4 . At 4 K, 1 is in the LS state and the bilayer cantilever shows a strong deflection. Under irradiation with a ~10-mW mm −2 unfocused laser beam (532 nm), one can observe the gradual decrease in the cantilever deflection until it reaches its initial form, corresponding to the fully HS form of the complex ( Supplementary Fig. S4a–f ). The absorption of green light by the LS complex leads to the population of the HS state, which persists (metastable) even after turning off the laser irradiation because of its very long lifetime at 4 K. Using a focussed laser beam to irradiate a section of a BSA of 1 at 78 K also resulted in deformation of the cantilever towards its initial high-spin form ( Supplementary Fig. S5 ). However, the light irradiation effect was not persistent after turning off the laser light because of the fast relaxation of the metastable HS state at this temperature. SCO/polymer composite bilayer actuators Polymer-based composite cantilevers were also constructed from an active SCO complex mixed with a polymer matrix and an inert layer of a different polymer as described in the Methods section. The SCO complexes used were Na 0.53 [Co 1.32 Fe(CN) 6 ]·4.4 H 2 O ( 2 ) (ref. 17 ), [Fe(Htrz) 2 (trz)]BF 4 ‘form b ’ ( 3 ) (ref. 18 ) and [Fe(Htrz) 2 (trz)]BF 4 ‘form a ’ ( 4 ) (ref. 18 ). The tip deflection of these composite cantilevers as a function of temperature is shown in Fig. 4 . Abrupt transitions with considerable hysteresis were observed, generating significant motion in these devices, as shown in Supplementary Fig. S6 . Good reproducibility of successive actuation cycles could be achieved after the initial thermal cycle ( Supplementary Fig. S7 ). 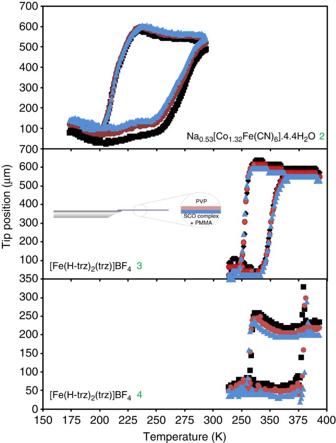Figure 4: Versatility of spin crossover bilayer actuators. These curves represent the behaviour of three cantilevers elaborated from SCO complex-PMMA composite films covered with PVP. Three different spin transition compounds were used to change the temperature of actuation. The displacements of the cantilever tips as a function of temperature are studied in three thermal cycles (squares are the first cycle, red circles are the second cycle, blue triangles are the third cycle). A schematic image representing the composite cantilevers is inset. The length of the cantilevers were 21.7, 34.1 and 43.6 mm. One may also note that in the case of the cantilever made from 4, a ‘spike’ appears around 380 K (see Figure 4 as well as Figure S7 ). We believe this well reproducible phenomenon is related to the glass transition of the PMMA, though more experiments will be necessary to clarify this question. Figure 4: Versatility of spin crossover bilayer actuators. These curves represent the behaviour of three cantilevers elaborated from SCO complex-PMMA composite films covered with PVP. Three different spin transition compounds were used to change the temperature of actuation. The displacements of the cantilever tips as a function of temperature are studied in three thermal cycles (squares are the first cycle, red circles are the second cycle, blue triangles are the third cycle). A schematic image representing the composite cantilevers is inset. The length of the cantilevers were 21.7, 34.1 and 43.6 mm. Full size image Whereas the length changes caused by NTE and SCO in free crystals of 1 are barely visible at the resolution of the microscope used, the macroscopic bending that those length changes cause in the BSA cantilever is considerable. The spontaneous strain along the c direction in 1 associated with the first-order spin transition is much greater than thermal expansion in the same temperature range, leading to the potential for extremely high-sensitivity thermomechanical actuation in properly designed SCO bilayers of 1 . The linear thermal expansion coefficient, α L , of the inert Al film is constant throughout the investigated temperature range, much larger than that of the c axis of the SCO crystal in the HS state and is opposite in sign ( α L =22.2 MK −1 and −2.7±0.7 MK −1 , respectively). The result is that on cooling from 343 to 95 K, the Al film contracts while the SCO crystal expands along the long axis; the differential thermal expansion of the two layers causes an upward bending of the crystal, as shown in Fig. 2d . On further cooling, the spontaneous strain associated with the spin transition causes the long axis of the SCO crystal to contract strongly, dwarfing the thermal contraction of the Al film and causing a substantial downward deflection of the cantilever ( Fig. 2e ). The opposite effects of thermal expansion and SCO on the crystal allow the separation of the two features, demonstrating unambiguously that amplified actuating motion may be produced purely as a product of SCO. Another important remark is that the hysteresis (shape memory) property encountered here (as well as in numerous SCO compounds) allows for power free force sustainability within the hysteresis range. By analogy to Timoshenko’s classical [19] classical thermomechanical model for bimetalic strips, we may see that the magnitude of cantilever deflection induced by NTE and SCO effects in 1 is dependent on the relative mechanical properties of each component, as well as on the cantilever geometry. In addition to the thermal expansion coefficients and magnitude of spontaneous strain induced by SCO, the aspect ratio of each layer, as well as their Young’s moduli, will affect the displacement of the cantilever tip. This model adapted to the case of SCO BSA actuators provides information useful for optimizing construction techniques as well as input for idealized geometries and component materials for fabrication at reduced length scales. Consider the classical case of curvature ( k ) of a rectangular bimetalic strip induced by the difference in thermal expansion coefficient of the two metals (mismatch of the strain) [16] : where Δ T is the temperature range of interest, E i is the Young’s modulus, a i is the height and α i is the linear thermal expansion coefficient of the i th material. It becomes clear that the important properties of the two layers that control the curvature are the relative Young’s moduli of the materials, their relative thickness (or height) and, of course, the mismatch of the strain in the temperature range of interest. We may approximate the path length ( δ ) travelled by the tip of the bimetal strip during bending (≈tip deflection if total path length is significantly shorter than the total strip length, L ) as a function of the curvature according to the following relationship: In the case of an SCO BSA actuator, the mismatch of the strain within the temperature range of the spin transition is a product of both the difference in thermal expansion of the SCO and inert layers and the expansion caused by the SCO in the active layer. As described previously, the many different known SCO compounds exhibit a diverse range of SCO behaviours, from first-order transitions that are complete in a few tenths of a Kelvin to very gradual crossovers that require several hundred Kelvin for complete HS→LS transition [14] , [15] . We may then estimate curvature as follows, by analogy to the general bimetal strip case: where L is the length of the long axis of the crystal and Δ L is the change in this length resulting from SCO. Taking into account the measured geometry of the two investigated cantilevers of 1 ( Table 1 ) and the Young’s modulus of aluminium metal ( E Al =69 GPa), we calculated the tip deflections related to the spin transition as a function of the Young’s modulus of 1 for these two actuators ( Fig. 5a ). The Δ L/L value related to the complete spin transition was extracted from the crystallographic measurements and used in these calculations. (An incomplete spin transition may occur in certain samples, leading to slightly different characteristics.) Table 1 Cantilever metrics. 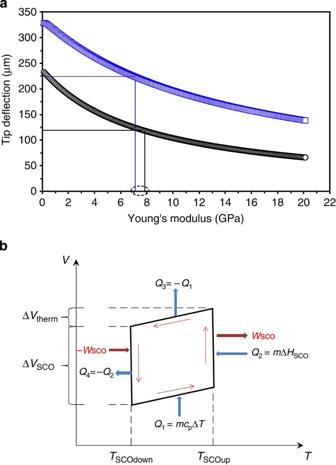Figure 5: Mechanical and thermodynamic properties of SCO BSAs. (a) Calculated tip deflections as a function of the Young’s modulus of1for BSA actuators consisting of a single crystal of1covered with a layer of Al. The experimentally determined tip deflections for two different cantilevers (open blue squares correspond to Cantilever A, open black circles correspond to Cantilever B) reveal a Young's Modulus of ~7−8 GPa. (b) Thermodynamic cycle in the V-T coordinates for a spin crossover actuator. Full size table Figure 5: Mechanical and thermodynamic properties of SCO BSAs. ( a ) Calculated tip deflections as a function of the Young’s modulus of 1 for BSA actuators consisting of a single crystal of 1 covered with a layer of Al. The experimentally determined tip deflections for two different cantilevers (open blue squares correspond to Cantilever A, open black circles correspond to Cantilever B) reveal a Young's Modulus of ~7−8 GPa. ( b ) Thermodynamic cycle in the V-T coordinates for a spin crossover actuator. Full size image As shown in Fig. 5a , the deflections that were experimentally observed for the two actuators allow us to extract the Young’s modulus of 1 with a fairly good precision. We can thus conclude that Young’s modulus of {Fe(3-CNpy)[Au(CN) 2 ] 2 }·2/3 H 2 O lies in the range of 7–8 GPa along the c-axis. For further calculations, the value of 7.5 GPa was used. (It may be worth noting that the Young’s modulus of the complex must be somewhat different in the two spin states. The value that is calculated above corresponds to the LS form as it was calculated from the curvature in this state.) One of the key parameters characterizing our actuators is the force generated via the spin transition. The reactive force at the end of a cantilever can be calculated as: where EI is the flexural rigidity. By taking into account the position of the centre of gravity in a bilayer beam, its flexural rigidity will be: where b is the width of the cantilever. For the two actuators of 1 that we studied in detail (see Table 1 ), these analytical calculations give the following reactive forces at the end of a cantilever: 2.7 × 10 −4 N ( A ) and 7.7 × 10 −4 N ( B ). To determine the energetic efficiency of our actuators, the volumetric work density must be first calculated. This describes the maximum mechanical work output per unit volume of an active material that drives actuation: where ε is a strain generated by SCO. For compound 1 , we obtained W / V =0.6 J cm −3 . This value is comparable to (or even higher than) the volumetric work that could be performed using piezoelectric ceramics and magnetostrictors [11] and is certainly a few orders higher than the work via a simple thermal expansion. For example, for the same complex 1 , a volumetric work density for a purely thermal actuation in a 5-K wide region (far from the spin transition) is ~0.0001 J cm −3 . The efficiency of the SCO actuator in one thermal cycle is shown in Fig. 5b and may be described as: For the actuation during the LS to HS switching in a complete thermal cycle, η is around 0.5% ( d =2.6 g cm −3 , Δ T =15 K, the specific heat capacity [14] c p was assumed to be 2 J g −1 K −1 and the enthalpy associated with the spin transition [14] Δ H SCO was assumed to be 20 J g −1 ). It should be noted that even if these SCO crystals have lower volumetric work density compared with shape-memory alloys (SMAs) or crystalline VO 2 (because of the higher Young’s modulus of these latter), SCO compounds perform well in terms of work efficiency because of the high spontaneous strain. The actuating cycle for this complex (15 K) is much smaller than for SMAs or VO 2 crystals (40 K) and is less affected by size-reduction effects (in case of SMAs, the memory effect starts to disappear at the submicrometric scale). Moreover, by changing the active compound to another SCO complex, the transition may become more abrupt or take place without any hysteresis loop. The transition temperature can be easily adjusted to the necessary region by changing the actuating complex or by specific physicochemical treatments including doping, for example. Using Equations 1, 2, 3, 4, 5, 6, it is possible to estimate the effect of modifying the BSA construction and hence to tune the deflection towards specific applications. For example, we may consider a BSA similar to the cantilever A , where L =876 μm, a SCO =21 μm, a Al =1 μm and Δ L/L =0.0126, with E Al =69 GPa and E SCO =7.5 GPa. By varying the thickness of the Al layer and by fixing the other parameters, we can calculate the tip deflection as a function of a Al . As shown in Fig. 6a , the highest tip deflection can be achieved using an ~4-μm thick Al layer; however, a significant cantilever deflection (for example, >100 μm) can be achieved for any thickness between 0.25 and 25 μm. 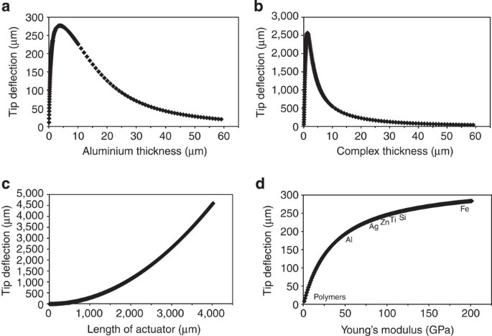Figure 6: Effect of modifying the cantilever construction on tip deflection. (a) The deflection of a cantilever of1depending on the thickness of the Al layer (aSCO=21 μm,LSCO=876 μm). (b) The deflection of a cantilever of1depending on the thickness of the SCO layer (aAl=1 μm,LSCO=876 μm). (c) The deflection of a cantilever of1as a function of its length (aAl=1 μm,aSCO=21 μm). (d) The deflection of a cantilever of1depending on the nature of the inert layer (aSCO=21 μm,ainert=1 μm,LSCO=876 μm). Figure 6: Effect of modifying the cantilever construction on tip deflection. ( a ) The deflection of a cantilever of 1 depending on the thickness of the Al layer ( a SCO =21 μm, L SCO =876 μm). ( b ) The deflection of a cantilever of 1 depending on the thickness of the SCO layer ( a Al =1 μm, L SCO =876 μm). ( c ) The deflection of a cantilever of 1 as a function of its length ( a Al =1 μm, a SCO =21 μm). ( d ) The deflection of a cantilever of 1 depending on the nature of the inert layer ( a SCO =21 μm, a inert =1 μm, L SCO =876 μm). Full size image In the same way, we have calculated the influence of the thickness of the SCO layer ( Fig. 6b ). As for the inert layer, the tip deflection as a function of the thickness of the SCO layer shows a maximum, which occurs in this case at about a SCO =1.3 μm. However, this thickness corresponds to an extremely high aspect ratio (~670), which would be difficult to obtain (for this compound) and would be certainly too fragile to be used in a practical device. Another parameter we investigated was the length of the actuator ( Fig. 6c ). In this case, a simple quadratic dependence is observed. However, very high aspect ratio crystals of 1 are neither easy to obtain nor simple to manipulate. Finally, we have also compared materials with different Young’s modulus for the inert layer ( Fig. 6d ). In case of highly rigid materials ( E =50–200 GPa), a large curvature could be achieved. This is not a case for the materials with less elevated elasticity modulus, for example, for organic polymers. That does not mean that such soft materials could not be used for these types of actuators, but rather it means that a different geometry of a cantilever is necessary (for example, with a thicker inert layer). While choosing the second material, the question of affinity between the two layers should be also taken in account. One major advantage of the BSA approach to harnessing the volume change during the spin transition is that it may be tuned to individual applications by using different SCO materials. To highlight the versatility of this approach, we have fabricated a series of composite materials consisting of various SCO complexes embedded in polymethylmethacrylate (PMMA). These composites were then used as the active layer for the BSA cantilevers, with the second, inert layer composed of Polyvinylpyrrolidone (PVP) (see insert in Fig. 4 and Supplementary Fig. S6 ). Three different SCO complexes were used to construct such composite cantilevers, each of which have different transition temperatures. By using other compounds from the vast number of known SCO-active systems, it is possible to tune the actuating conditions of the actuator device using this simple and highly versatile approach. However, as size decreases, the methods used here for the construction of cantilevers and the detection of motion become increasingly less suitable. Clearly, the development of micro- and nano-scale fabrication protocols for parallel synthesis of these materials is required to adapt this concept to practical applications at reduced length scales. In this context, the polymer/SCO composites offer interesting perspectives, as the methods for processing polymeric materials (including composites) in MEMS/NEMS (micro- or nano-electromechanical systems) applications are already very well developed; crucially the retention of SCO properties as size decreases to the nano-scale has been clearly demonstrated [20] and recently even imaged in a single particle [21] . The appropriate choice of the SCO compound can produce an actuator with different characteristics tailored to the desired application; the abruptness of the transition, accessible strain, efficiency, shape-memory properties or sensitivity to chemical vapours and so on are the features specific to each compound. We anticipate that this approach to the conversion of thermal, electromagnetic, chemical and mechanical energies into useful motion at the nano-scale using SCO systems will open up a new direction in research into functional molecular materials. Chemical synthesis SCO BSAs of 1 —needle-like tetragonal single crystals of the 3D SCO coordination polymer {Fe(3-CNpy)[Au(CN) 2 ] 2 }·2/3 H 2 O ( 1 ), where py=pyridine—were synthesized in a similar manner to that previously described [16] . FeCl 2 ·4 H 2 O (10 mg, 0.05 mmol), 3-cyanopyridine (23 mg, 0.22 mmol) and KAu(CN) 2 (28.7 mg, 0.1 mmol) were dissolved in 6 ml of MeOH/H 2 O and stirred for an hour at room temperature. The solution was left open to air to crystallize. After ~1 week, a mixture of crystalline forms was observed as previously reported [16] . After further standing for ~4 weeks, the only crystals observed were the needle-like crystals of 1 . Microcrystaline SCO complexes of Na 0.53 [Co 1.32 Fe(CN) 6 ]·4.4 H 2 O ( 2 ) (ref. 17 ), [Fe(Htrz) 2 (trz)]BF 4 ‘form b ’ ( 3 ) (ref. 18 ) and [Fe(Htrz) 2 (trz)]BF 4 ‘form a ’ ( 4 ) (ref. 18 ) were prepared according to literature methods for use in the polymer composite cantilevers. Cantilever construction from single crystals of 1 In general, a cylindrical graphite rod with a diameter of ~750 μm was tapered to a point at one end. A small amount of epoxy resin glue was added to the tapered rod. A single needle-shaped crystal of 1 was set into the epoxy resin and allowed to dry. The cantilever was then coated with a 5-nm film of Ti and a 1-μm film of Al by thermal evaporation in vacuum. Construction of polymer/SCO composite cantilevers In general, a microcrystalline powder of the SCO compound (2 mg) was disaggregated with ultrasonic treatment and mechanically dispersed in a solution of PMMA 550,000 (2 mg) in CHCl 3 (100 μl). This dispersion was deposited on a silicon substrate (1 cm 2 ) and dried in air. In the next step, a solution of PVP 40,000 (0.5 mg) in absolute EtOH (25 μl) was layered over the composite film. After the evaporation of the ethanol, the bilayer film was carefully removed from the substrate and manually cut into cantilevers. They were fixed on hypodermic needles with a cyanoacrylic glue. The thickness of the active layer is ~20–25 μm, whereas the PVP layer is ~4 μm. By changing the concentrations and the deposited volume, one can easily adjust the thickness of the layers. The choice of PMMA and PVP was mainly dictated by solvent compatibilities; however, other factors must be also considered, such as the occurrence of phase transitions or the ability to form continuous films. Single-crystal X-ray diffraction Variable temperature single-crystal X-ray diffraction data represented in Fig. 1a of the main text were collected on a Bruker ApexII diffractometer. Temperature was controlled using an open-flow nitrogen gas cooling device. Cell parameters were determined from raw diffraction images and refined using the ApexII software. Raman spectroscopy Variable temperature Raman spectra were acquired by means of a LabramHR (Horiba Jobin Yvon) micro-spectrometer in conjunction with a THMS600 liquid-nitrogen cryostage (Linkam Scientific Instruments). Raman scattering was excited using either a HeNe (632.8 nm) or a Nd:YAG (532 nm) laser. The excitation power on the sample was set to 0.01 mW and the absence of noticeable laser-heating effects was carefully tested. The laser beam was focused on the crystals via a × 50 long-working-distance objective (NA=0.45, WD=15 mm), which also served to collect the scattered photons. The Rayleigh scattering was removed by a holographic notch filter and the Raman spectra were recorded with acquisition times of 120 s. Several spectral features were found to be attributable to the spin-state change; however, we have chosen to follow the strong intensity CN stretching modes, with a characteristic HS and LS marker around 2,188 and 2,192 cm −1 , respectively (see Supplementary Fig. S4 ). For instrumental reasons (better spectral resolution and higher intensity), most experiments were carried out at 633 nm excitation; however, the main findings were confirmed by the 532 nm excitation as well. As shown in Fig. 3b , the intensity ratio of the LS and HS CN stretching modes allows the reproduction of the thermal spin transition, which occurs around 120 K. One shall note that the completeness of the SCO, the transition temperature as well as the hysteresis width were found to vary slightly from one crystal to another. This is a well-known feature of first-order phase transitions, where intrinsic crystal defects are known to have a strong influence on the phase transformation kinetics [22] . Upon cooling to 78 K, a return to the HS state is inferred from the Raman spectra, which we can attribute to the well-known LIESST effect [14] , [15] . This LS to HS photoswitching phenomenon was observed using both red and green laser excitations, with the latter providing better conversion efficiency ( Supplementary Fig. S4 ). An important point to note here is that at 90 K the system returns to a fully LS state. This is obviously not possible if the HS fraction at 78 K is generated by laser-induced heating, thus providing irrefutable proof for a genuine photo-induced spin-state switching at 78 K. Optical microscopy Variable temperature optical microscopy images of the free and cantilevered crystals were recorded in bright- or dark-field reflection mode using an Olympus BX51 microscope equipped with a megapixel format charge-couple device (CCD, Ikon-M Andor Technology) and a × 5 objective. The sample temperature was controlled using a Linkam THMS600 cryo-stage (in dry N 2 atmosphere). Between 343 and 143 K, heating and cooling rates were 5 K min −1 and images were taken every 12 s (every 1 K). Between 143 and 78 K, heating and cooling rates were 2 K min −1 and images were taken every 7.5 s (every 0.25 K). During the thermal cycles, the sample was illuminated with a halogen lamp (400–700 nm). Supplementary Movie 1 of one of the BSAs switching during a single 50-K min −1 cooling and heating cycle between 113 and 78 K was also recorded using the colour CCD and is presented in Supplementary Movie 1. Photoswitching experiments were carried out at 78 K using the Raman spectroscopy setup and a colour CCD. The frequency doubled line (532 nm) of a Nd:YAG laser was focused on the cantilever by an × 5 microscope objective, and the images were acquired while the laser was turned on/off successively. In other experiments ( vide infra ), the cantilever was exposed to the unfocused laser light at 4 K and images were acquired before and after the laser exposure. In all microscopy experiments, the sample temperature was controlled using a Linkam THMS600 cryo-stage (in dry N 2 atmosphere). We shall point out, however, that for obvious reasons the real temperature of a crystal, placed directly on the cold finger of the cryostat, and that of a cantilever, attached only at one of its extremities, will be different. In addition, as mentioned previously, slight intrinsic variations from sample to sample may occur in the transition temperatures of individual crystals. Moreover, the presence of the Al layer may also slightly influence the spin transition in the composite BSAs. For all these reasons, the comparison of the exact transition temperature of free and cantilevered crystals is meaningless. Furthermore, in some cases a graphite support was used to adjust the orientation of the graphite rod and bring the BSA into focus. Despite this, the variation of the SCO temperature between free crystals and BSAs was no more than 30 K. Light-induced actuation of a cantilever A cantilever of 1 was also used to demonstrate a possibility of actuation induced by light irradiation. The sample was cooled down to 4 K, which was accompanied by a typical cantilever deflection related to the thermal spin transition ( Supplementary Fig. S6 a→c). The cantilever was then exposed to an ~10-mW/mm 2 unfocused laser beam (532 nm). Under light irradiation, one can observe the gradual decrease in the cantilever deflection until it reaches its initial form, corresponding to the fully HS form of the complex ( Supplementary Fig. S6 d→f). Indeed, the absorption of green light by the LS complex leads to the population of the HS state, which persists (metastable) even after turning off the laser irradiation because of its very long lifetime at 4 K. We have also carried out a series of experiments at 78 K using the same experimental setup; however, in this case we had to focus the laser light on the cantilever using a × 5 objective. As shown in Supplementary Fig. S5 , in this case also we observed the deformation of the cantilever towards the initial form (HS state). However, the light irradiation effect was not persistent after turning off the laser light—owing to the fast relaxation of the metastable HS state at this temperature. Image treatment So as to give a rigorous analysis for the deflection of the tip, we developed an image registration routine under MATLAB environment employing the Image Processing Toolbox software. Image registration is the process of aligning two or more images of the same scene. Our routine compensates automatically for any drift of the sample obtained during the experiments. It receives a stack of images (in the TIFF format) and asks from the user two inputs: (i) a section of interest or feature in the first image of the stack that will be tracked during the alignment process and (ii) at least three reference points (it could be more) present in all the images of the stack (as the sample drifts, there are some regions of the image that may appear/disappear from the field of view) that would be used later for fine tuning of the alignment. For our experiments, we selected as a feature the graphite rod of the cantilever; this section can be easily tracked and its shape will not be dramatically affected during the thermal cycles, contrary to the body of the cantilever. Moreover, the reference points were selected on this area to avoid the bending effects in the cantilever. Once these parameters are defined by the user, the routine executes the function of, what is called in signal processing, normalized 2D cross-correlation between the feature and the rest of the images of the stack following Equation 11 [23] : where CCR(u, v) is the cross-correlation, f(x, y) is the image to be analysed, t is the feature, is the mean value of the selected feature and u,v is the mean value of f(x, y) in the region under the feature. The cross-correlation is a measure of the similarity of two waveforms as a function of a parameter-lag (time, space, frequency and so on) applied to one of them. In our case, this procedure can be understood as a spatial sweep of the feature over a given image seeking the place of maximum similitude. Thus, a preliminary set of offset values for X and Y can be inferred from each cross-correlation. However, this operation does not take into account the slight rotations that the sample has during the experiment (it involves only translation); as a result, we have the stack of images closely aligned but they do not match exactly. To solve this, the routine uses a punctual cross-correlation in the vicinity of the coordinates of the reference points in each pre-aligned image searching for the real positions of the reference points. With this information, the routine can establish a spatial transformation for each image of the stack in order to match them with the first image of the experiment. Once all images of an experiment were registered in this manner, the ImageJ software was used to analyse the deflection of the tip. Given the long radius of the curvature, we assumed that the path travelled by the tip of the cantilevers could be described by a straight line during deflection. Thus, a line of reference, with which the tip of the cantilever was always in contact was drawn, and the intensity profile along this line was plotted for each image. In these profiles, the minimum corresponds to the tip of the cantilever; consequently, by plotting the relative position of this minimum as a function of temperature we can quantify its deflection. How to cite this article: Shepherd, H. J. et al . Molecular actuators driven by cooperative spin-state switching. Nat. Commun. 4:2607 doi: 10.1038/ncomms3607 (2013).